Cholinergic pesticides cause mushroom body neuronal inactivation in honeybees Pesticides that target cholinergic neurotransmission are highly effective, but their use has been implicated in insect pollinator population decline. Honeybees are exposed to two widely used classes of cholinergic pesticide: neonicotinoids (nicotinic receptor agonists) and organophosphate miticides (acetylcholinesterase inhibitors). Although sublethal levels of neonicotinoids are known to disrupt honeybee learning and behaviour, the neurophysiological basis of these effects has not been shown. Here, using recordings from mushroom body Kenyon cells in acutely isolated honeybee brain, we show that the neonicotinoids imidacloprid and clothianidin, and the organophosphate miticide coumaphos oxon, cause a depolarization-block of neuronal firing and inhibit nicotinic responses. These effects are observed at concentrations that are encountered by foraging honeybees and within the hive, and are additive with combined application. Our findings demonstrate a neuronal mechanism that may account for the cognitive impairments caused by neonicotinoids, and predict that exposure to multiple pesticides that target cholinergic signalling will cause enhanced toxicity to pollinators. Pesticide exposure is a potential contributor to the current decline in populations of pollinating insects, which provide essential pollination services for food production [1] . In the past 20 years, there has been a rapid increase in the use of neonicotinoids [2] , systemic insecticides with improved selectivity for insects relative to vertebrates [3] . However, non-target pollinators may be adversely affected via consumption of contaminated nectar and pollen [4] , [5] , [6] . A growing number of laboratory and field studies have shown that exposure of bees to sublethal levels of neonicotinoids results in behavioural changes that impact on survival, including impairment of learning and memory, disrupted navigation and reduced foraging activity [7] , [8] , [9] , [10] , [11] . Furthermore, the effects of neonicotinoids may be exacerbated by coexposure to other pesticides [11] , [12] , such as the miticides used by beekeepers to combat Varroa infestations, which are the major chemical contaminants of honeybee hives [13] , [14] . Interactions between pesticides are possible at multiple levels, for example, via competition for metabolic enzymes [15] and cellular efflux [16] , but interactions at their pharmacological target sites have not been reported. Both neonicotinoids and organophosphates, such as the miticide coumaphos, target cholinergic signalling, which comprises the majority of excitatory neurotransmission in the insect central nervous system [17] . Neonicotinoids acts as nicotinic acetylcholine (ACh) receptor (nAChR) agonists, whereas organophosphates inhibit acetylcholinesterase (AChE), which terminates the action of synaptically released ACh at both nicotinic and muscarinic receptors. The neonicotinoid imidacloprid has been shown to be a partial agonist of nAChRs in dissociated honeybee Kenyon cells (KCs) in culture [18] , [19] , which are the major neuronal component of the mushroom bodies and comprise over 40% of neurons in the honeybee brain [20] . The mushroom bodies are a higher-order insect brain structure that mediates multisensory integration, learning and memory [21] , [22] , cognitive functions that are disrupted by neonicotinoids [7] , [8] . However, the effect of prolonged activation of native nAChRs by cholinergic pesticides on KC function is not known. Our recent development of a technique to make whole-cell recordings from KCs in acutely isolated honeybee brain enables the effect of cholinergic pesticides on the function of KCs to be determined. This technique provides significant advantages over cultured KC recordings for assessing the neurophysiological consequences and concentration dependence of neonicotinoid effects, including native connectivity and nAChR expression. Furthermore, recordings in intact tissue are essential for investigating the effect of organophosphates, which are dependent on the intact synaptic architecture. We find that two widely used neonicotinoids (imidacloprid and clothianidin) and the active metabolite of coumaphos (coumaphos oxon) have pronounced effects on KC excitability and nAChR-mediated responses at nanomolar concentrations, and that the neonicotinoid and miticide effects are additive at the neuronal level. The results provide a cellular mechanism for the observed cognitive impairment of bees by neonicotinoids, and suggest that a similar detrimental effect may arise from chronic exposure to coumaphos when used as an in-hive miticide to control Varroa infestations. In addition, these findings indicate that coexposure to cholinergic pesticides with different mechanisms of action will be particularly detrimental to honeybee fitness. Membrane properties of KCs in honeybee brain Whole-cell recordings were made from KCs in acutely isolated honeybee brain. KC somata are easily identified as the numerous, tightly packed cells, with a diameter of 5–10 μm within the mushroom body calyces ( Fig. 1a ) [23] . The identity of the recorded neurons was confirmed by measuring their passive and active membrane properties. KCs in intact honeybee brain have a membrane capacitance ( C M ) of 3.6±0.2 pF and input resistance ( R I ) of 2.8±0.2 GΩ ( n =183), similar to that of cultured honeybee KCs [24] and to morphologically identified KCs in the intact cockroach brain [25] . Depolarizing voltage steps evoke membrane currents ( I M ) that display time- and voltage-dependent characteristics of voltage-gated Na + channels and A-type, delayed rectifier and Ca 2+ -activated K + channels, as observed in cultured KCs ( Fig. 1c ) [26] , [27] , [28] , [29] . Under current clamp, resting membrane potential ( V M ) is −62±1 mV ( n =22). Current injection evokes action potential (AP) firing that exhibits strong adaptation in frequency ( Fig. 1d ). This AP frequency adaptation is largely absent from cultured honeybee KCs [29] but is similarly pronounced in KCs in intact cockroach brain [25] , reinforcing the importance of studying intact tissue. 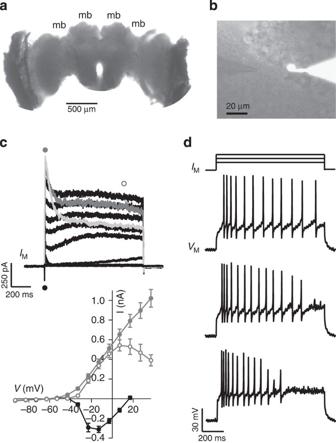Figure 1: Kenyon cell recordings in acutely isolated honeybee brain. (a,b) Images of an acutely isolated honeybee brain (mb, mushroom body) and a KC whole-cell recording with the fluorescent dye Lucifer Yellow in the patch electrode; to the left is a second micropipette used for pressure application of ACh. (c) Top, the current response to voltage steps (10 mV increments from a holding potential of −73 mV) showing activation of inward Na+and outward K+currents. Below, mean (±s.e.m.)I/Vrelationships (n=11) for the peak inward current (black circle), peak outward current (grey circle) and sustained outward current (open circle). The N-shape of theI/Vrelationship (open circle) indicates that Ca2+-activated K+channels contribute to the sustained current25,26. (d) Under current clamp, current injection (+20–+40 pA) evokes AP firing that exhibits adaptation in both frequency and amplitude, and a short delay between the current step and the first AP. Repetitive AP firing is therefore inhibited by sustained depolarization. Figure 1: Kenyon cell recordings in acutely isolated honeybee brain. ( a , b ) Images of an acutely isolated honeybee brain (mb, mushroom body) and a KC whole-cell recording with the fluorescent dye Lucifer Yellow in the patch electrode; to the left is a second micropipette used for pressure application of ACh. ( c ) Top, the current response to voltage steps (10 mV increments from a holding potential of −73 mV) showing activation of inward Na + and outward K + currents. Below, mean (±s.e.m.) I / V relationships ( n =11) for the peak inward current (black circle), peak outward current (grey circle) and sustained outward current (open circle). The N-shape of the I / V relationship (open circle) indicates that Ca 2+ -activated K + channels contribute to the sustained current [25] , [26] . ( d ) Under current clamp, current injection (+20–+40 pA) evokes AP firing that exhibits adaptation in both frequency and amplitude, and a short delay between the current step and the first AP. Repetitive AP firing is therefore inhibited by sustained depolarization. Full size image Neonicotinoids depolarize KCs Cholinergic pesticides were bath-applied at low concentrations to simulate environmental exposure to field-relevant concentrations found in crop pollen and nectar [8] , and within hives [14] . KCs were recorded under current clamp at resting V M to determine the effect of the pesticides on membrane excitability and AP firing. The neonicotinoid clothianidin (1–100 nM, n =8) evokes a rapid, concentration-dependent depolarization of KC V M ( Fig. 2a ). The depolarization is reversed by the nAChR antagonist d-tubocurarine (d-TC, 500 μM, n =3; Fig. 2a ), showing that it is due to sustained nAChR activation by the neonicotinoids. AP firing occurs during the initial development of the depolarization but not during the plateau phase ( Fig. 1b ), reflecting the properties of AP frequency adaptation in KCs ( Fig. 1d ). The neonicotinoid imidacloprid (10–500 nM, n =7) and imidacloprid–olefin (50–500 nM, n =4), a major metabolite that also acts as a nAChR agonist [30] , similarly evoke sustained depolarization of KC V M that is reversed by d-TC ( Fig. 2e ). At 10 nM, clothianidin evokes a significantly larger depolarization than imidacloprid ( n =3-4, P <0.05), consistent with their respective actions as full and partial nAChR agonists [31] , [32] . 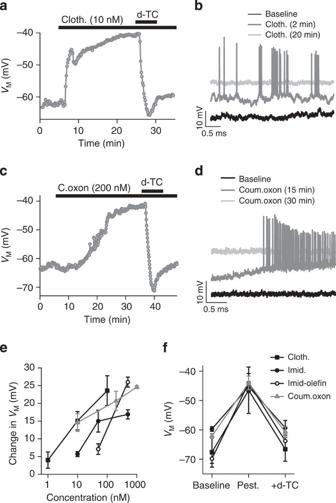Figure 2: Cholinergic pesticides depolarize KCs at low concentrations. The effect of neonicotinoids and coumaphos oxon on KC membrane potential (VM) and AP firing were investigated under current clamp. (a) Bath application of clothianidin evokes sustained depolarization of KCVM. Coapplication of the nAChR antagonist d-TC (500 μM, here and subsequently) reverses the depolarization, indicating that it is mediated by nAChR activation. (b) AP firing is transiently observed during the development of the depolarization (2 min after clothianidin application), but is inhibited during the subsequent sustained depolarization (20 min example trace). (c) Coumaphos oxon evokes a more slowly developing depolarization of KCVM, which is reversed by d-TC. The slower time course is consistent with nAChR activation by accumulated ACh as a result of AChE inhibition. (d) AP firing is again transiently observed during the development of the depolarization (15 min after coumaphos oxon application) but not during the sustained phase (30 min example trace). (e) Dose dependence of the mean (±s.e.m.) depolarizing effects of the neonicotinoids clothianidin (black square,n=4) and imidacloprid (black circle,n=3-4), the metabolite imidacloprid–olefin (open circle,n=4) and the organophosphate coumaphos oxon (grey triangle,n=2–7;nnumbers refer to each data point; for all data points ≥10 nM,P<0.05, pairedt-test). (f) Mean (±s.e.m.) data showing the reversal by d-TC of the depolarizations evoked by clothianidin (10–100 nM,n=3), imidacloprid (50–500 nM,n=4), imidacloprid–olefin (500 nM,n=3) and coumaphos oxon (200 nM–1 μM,n=4). All four pesticides potently modulate KC excitability by causing sustained activation of nAChRs. Figure 2: Cholinergic pesticides depolarize KCs at low concentrations. The effect of neonicotinoids and coumaphos oxon on KC membrane potential ( V M ) and AP firing were investigated under current clamp. ( a ) Bath application of clothianidin evokes sustained depolarization of KC V M . Coapplication of the nAChR antagonist d-TC (500 μM, here and subsequently) reverses the depolarization, indicating that it is mediated by nAChR activation. ( b ) AP firing is transiently observed during the development of the depolarization (2 min after clothianidin application), but is inhibited during the subsequent sustained depolarization (20 min example trace). ( c ) Coumaphos oxon evokes a more slowly developing depolarization of KC V M , which is reversed by d-TC. The slower time course is consistent with nAChR activation by accumulated ACh as a result of AChE inhibition. ( d ) AP firing is again transiently observed during the development of the depolarization (15 min after coumaphos oxon application) but not during the sustained phase (30 min example trace). ( e ) Dose dependence of the mean (±s.e.m.) depolarizing effects of the neonicotinoids clothianidin (black square, n =4) and imidacloprid (black circle, n =3-4), the metabolite imidacloprid–olefin (open circle, n =4) and the organophosphate coumaphos oxon (grey triangle, n =2–7; n numbers refer to each data point; for all data points ≥10 nM, P <0.05, paired t -test). ( f ) Mean (±s.e.m.) data showing the reversal by d-TC of the depolarizations evoked by clothianidin (10–100 nM, n =3), imidacloprid (50–500 nM, n =4), imidacloprid–olefin (500 nM, n =3) and coumaphos oxon (200 nM–1 μM, n =4). All four pesticides potently modulate KC excitability by causing sustained activation of nAChRs. Full size image Coumaphos oxon depolarizes KCs Coumaphos is inactive as an AChE inhibitor and requires metabolic conversion to its active form, coumaphos oxon, which is a potent AChE inhibitor ( Fig. 3 ) [33] . Bath application of coumaphos oxon (10 nM–1 μM, n =12) to current-clamped KCs evokes a concentration-dependent depolarization of V M ( Fig. 2c ). The depolarization is reversed by d-TC ( n =4; Fig. 2c ), confirming that it is mediated by sustained nAChR activation. As with the neonicotinoids, AP firing is observed during the development of the depolarization but not during the sustained phase ( Fig. 2d ). However, the depolarization evoked by coumaphos oxon develops more slowly ( Fig. 2c ), consistent with nAChR activation by the accumulation of endogenous ACh as a result of AChE inhibition. Thus, prolonged activation of nAChRs, either directly by neonicotinoids or indirectly by coumaphos oxon, disrupts KC function by causing a transient increase in excitability followed by a depolarization-block of AP firing, due to the properties of voltage-gated Ca 2+ and Ca 2+ -activated K + currents in KCs [25] . 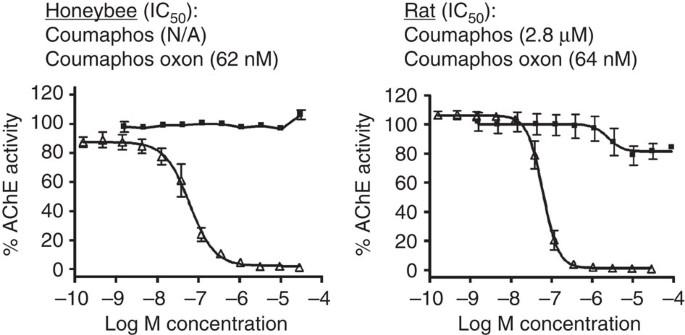Figure 3: Coumaphos oxon potently inhibits AChE. Mean (±s.e.m.) AChE activity measured in honeybee brain (n=3) and rat brain (n=3) by the Ellman assay, showing inhibition by coumaphos oxon but little effect of coumaphos. AChE activity was normalized to control measurements; IC50values were obtained from Hill equation fits of the data. Figure 3: Coumaphos oxon potently inhibits AChE. Mean (±s.e.m.) AChE activity measured in honeybee brain ( n =3) and rat brain ( n =3) by the Ellman assay, showing inhibition by coumaphos oxon but little effect of coumaphos. AChE activity was normalized to control measurements; IC 50 values were obtained from Hill equation fits of the data. Full size image ACh-evoked responses in KCs in honeybee brain To determine the effect of cholinergic pesticides on transient nAChR-mediated responses, ACh was pressure-applied (200 μM, 100 ms duration, 30 s intervals) from a second micropipette positioned close to the recorded KC ( Fig. 1b ). Exogenous ACh was used to activate nAChRs, as electrically evoked synaptic currents are difficult to record in this preparation. Under voltage clamp, ACh evokes transient inward currents ( Fig. 4a , I M trace) that exhibit a reversal potential of approximately −20 mV and a slight inward rectification ( n =5; Fig. 4c ). Under current clamp, ACh evokes transient membrane depolarization of 15±1 mV ( n =9) that is normally associated with a burst of APs ( Fig. 4a , V M trace). ACh-evoked currents are fully inhibited by the nAChR antagonists d-TC (500 μM, n =5) and α-bungarotoxin (1–5 μM, n =5; Fig. 4a ), indicating that muscarinic receptors do not contribute to the response, as found previously in cultured KCs [24] , [34] . However, ACh-evoked currents exhibit considerable variability in size and kinetics between KCs in intact tissue ( Fig. 4d ), which is not seen in cultured KCs [19] , [24] , [34] . This variability in intact mushroom body KC ACh responses may result from the differential expression of fast and slow desensitizing nAChR subtypes [19] , [24] , [35] , [36] . 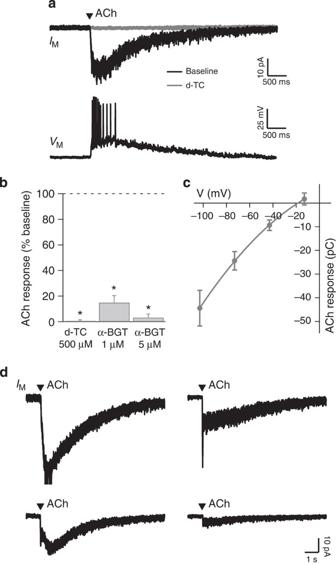Figure 4: Properties of KC ACh responses. (a) Local application of ACh (200 μM, 100 ms) to a voltage-clamped KC evokes a transient inward current that is blocked by bath application of d-TC, indicating that it is solely mediated by nAChRs. In the same KC under current clamp, ACh evokes a transient depolarization and a burst of APs (shown below). (b) Mean (±s.e.m.) data showing the inhibition of ACh-evoked currents by d-TC (n=5) and by α-bungarotoxin (α-BGT;n=5), which inhibits vertebrate α7 nAChRs (*P<0.05, pairedt-test). (c) Mean (±s.e.m.) response size at different holding potentials, showing that the voltage-dependence of ACh responses exhibits slight inward rectification (n=5). (d) Example ACh responses showing the variability in amplitude and kinetics of the response between KCs, with distinct fast and slow components in some recordings. Figure 4: Properties of KC ACh responses. ( a ) Local application of ACh (200 μM, 100 ms) to a voltage-clamped KC evokes a transient inward current that is blocked by bath application of d-TC, indicating that it is solely mediated by nAChRs. In the same KC under current clamp, ACh evokes a transient depolarization and a burst of APs (shown below). ( b ) Mean (±s.e.m.) data showing the inhibition of ACh-evoked currents by d-TC ( n =5) and by α-bungarotoxin (α-BGT; n =5), which inhibits vertebrate α7 nAChRs (* P <0.05, paired t -test). ( c ) Mean (±s.e.m.) response size at different holding potentials, showing that the voltage-dependence of ACh responses exhibits slight inward rectification ( n =5). ( d ) Example ACh responses showing the variability in amplitude and kinetics of the response between KCs, with distinct fast and slow components in some recordings. Full size image Neonicotinoids inhibit KC ACh responses The effects of neonicotinoids on baseline I M and ACh-evoked currents were investigated in voltage-clamped KCs. Bath application of imidacloprid (50 nM–10 μM; n =25) evokes a tonic inward current in KCs, observed as an increase in the amplitude and variance of I M ( Fig. 5a–e ). The tonic current exhibits a variable degree of desensitization (for example, present in Fig. 5b but absent in Fig. 5c ), and is blocked by d-TC ( n =3; Fig. 5c ). This effect of imidacloprid is consistent with the sustained activation and desensitization of KC nAChRs. As a result, imidacloprid inhibits ACh-evoked responses ( Fig. 5a ). A dose–response plot of ACh response inhibition by imidacloprid yields an IC 50 value of 295 nM ( Fig. 5f ). Clothianidin (200 nM; n =3) similarly evokes a tonic inward current and inhibits ACh responses ( Fig. 5e ). Neonicotinoids, therefore, reduce KC responsiveness to ACh. 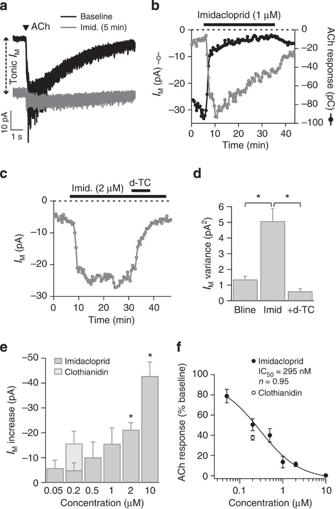Figure 5: Neonicotinoids evoke a tonic nAChR current and inhibit ACh responses. The effect of neonicotinoids on baselineIMand on ACh responses were investigated under voltage clamp. (a) Bath application of imidacloprid (1 μM) evokes an inward shift in the baseline current (tonicIM) and inhibits responses evoked by local application of ACh (200 μM, 100 ms). (b) The time course of the effect of imidacloprid onIM(○) and ACh responses (). The tonic current (increase inIM) develops rapidly and then declines slowly due to nAChR desensitization; ACh responses are rapidly inhibited and remain inhibited for the duration of imidacloprid application. (c) In a different KC, imidacloprid evokes a tonic current that exhibits little desensitization. Coapplication of d-TC reverses the tonic current, showing that it is due to sustained nAChR activation. (d) Mean (±s.e.m.) data showing that imidacloprid (pooled 1–10 μM) also evokes an increase inIMvariance (current noise;n=16, *P<0.01, pairedt-test) that is reversed by d-TC (2 μM imidacloprid,n=3, *P<0.05, unpairedt-test), consistent with increased nAChR channel activity. (e) The dose dependence of the peak tonic current evoked by imidacloprid (mean±s.e.m.,n=3–7 for each concentration, *P<0.05, pairedt-test) and the effect of clothianidin (200 nM,n=3) for comparison. (f) The dose dependence of ACh response inhibition by imidacloprid (mean±s.e.m.,n=3–7) with a Hill equation fit, and the effect of clothianidin (200 nM,n=3) for comparison. ACh response inhibition was measured after at least 10 min of neonicotinoid application. The neonicotinoids reduce KC responsiveness to ACh by tonically activating and desensitizing nAChRs. Figure 5: Neonicotinoids evoke a tonic nAChR current and inhibit ACh responses. The effect of neonicotinoids on baseline I M and on ACh responses were investigated under voltage clamp. ( a ) Bath application of imidacloprid (1 μM) evokes an inward shift in the baseline current (tonic I M ) and inhibits responses evoked by local application of ACh (200 μM, 100 ms). ( b ) The time course of the effect of imidacloprid on I M ( ○ ) and ACh responses ( ). The tonic current (increase in I M ) develops rapidly and then declines slowly due to nAChR desensitization; ACh responses are rapidly inhibited and remain inhibited for the duration of imidacloprid application. ( c ) In a different KC, imidacloprid evokes a tonic current that exhibits little desensitization. Coapplication of d-TC reverses the tonic current, showing that it is due to sustained nAChR activation. ( d ) Mean (±s.e.m.) data showing that imidacloprid (pooled 1–10 μM) also evokes an increase in I M variance (current noise; n =16, * P <0.01, paired t -test) that is reversed by d-TC (2 μM imidacloprid, n =3, * P <0.05, unpaired t -test), consistent with increased nAChR channel activity. ( e ) The dose dependence of the peak tonic current evoked by imidacloprid (mean±s.e.m., n =3–7 for each concentration, * P <0.05, paired t -test) and the effect of clothianidin (200 nM, n =3) for comparison. ( f ) The dose dependence of ACh response inhibition by imidacloprid (mean±s.e.m., n =3–7) with a Hill equation fit, and the effect of clothianidin (200 nM, n =3) for comparison. ACh response inhibition was measured after at least 10 min of neonicotinoid application. The neonicotinoids reduce KC responsiveness to ACh by tonically activating and desensitizing nAChRs. Full size image Coumaphos oxon has a biphasic effect on KC ACh responses The effect of coumaphos oxon on baseline I M and ACh responses was also investigated, and was found to be distinct from that of neonicotinoids. Bath application of coumaphos oxon (50 nM–1 μM; n =11) initially potentiates ACh responses ( Fig. 6a ), consistent with inhibition of AChE activity. However, with continued exposure to coumaphos oxon, a tonic inward current develops that is reversed by d-TC ( n =4; Fig. 6a ), indicating sustained nAChR activation by endogenous ACh. Importantly, the tonic current is associated with an inhibition of ACh-evoked responses ( Fig. 6a ). Thus, coumaphos oxon exerts a biphasic effect of on KC ACh responses: initial potentiation followed by inhibition. Furthermore, the time required to reach the peak potentiation and subsequent inhibition of ACh responses is dependent on the concentration of coumaphos oxon ( Fig. 6e ). The potentiation and inhibition occur more rapidly with higher doses, indicating that both the level and duration of exposure to coumaphos oxon will determine its effects on KC function. For comparison, we tested the effect of the widely used organophosphate AChE inhibitor donepezil and the inactive parent compound coumaphos. Donepezil (10–100 μM, n =7) has similar effects on ACh responses and I M as coumaphos oxon ( Fig. 6c ), but coumaphos (1–50 μM, n =10) does not. However, at concentrations ≥10 μM, coumaphos appears to directly inhibit nAChRs ( Fig. 6f–h ), an effect that has also been observed with other organophosphates [37] . 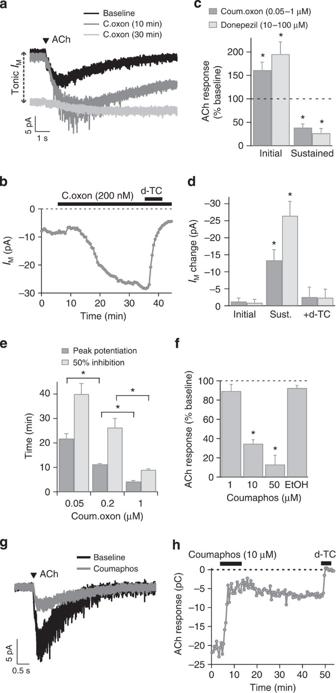Figure 6: Coumaphos oxon has a biphasic effect on ACh responses. The effects of coumaphos oxon on baselineIMand ACh responses were investigated under voltage clamp. (a) Coumaphos oxon (200 nM) initially potentiates ACh responses (10 min after application), consistent with AChE inhibition. Subsequently, coumaphos oxon evokes a tonic current and inhibits ACh responses (30 min after application). (b) The time course of the effect of coumaphos oxon onIMin a different KC. The tonic current develops slowly and is reversed by d-TC, consistent with nAChR activation by accumulated endogenous ACh. (c) Mean (±s.e.m.) data showing the biphasic effect (initial potentiation followed by sustained inhibition) of coumaphos oxon (n=11, *P<0.01, pairedt-test) on ACh responses. Included for comparison is the effect of the widely used AChE inhibitor donepezil (n=7, *P<0.01, pairedt-test). (d) Mean (±s.e.m.) data showing the effects of coumaphos oxon (n=11) and donepezil (n=7) onIM(*P<0.01, pairedt-test). Inhibition of ACh responses is associated with an increase inIM(tonic current). (e) Mean (±s.e.m.) data showing that the time course of the biphasic effect of coumaphos oxon on ACh responses is dependent on concentration (0.05 μM,n=4; 0.2 μM,n=3; 1 μM,n=4; *P<0.01, unpairedt-test). (f) Mean (±s.e.m.) data showing that the parent compound coumaphos inhibits ACh responses at concentrations ≥10 μM (1 μM,n=3; 10 μM,n=5; 50 μM,n=3; *P<0.05, pairedt-test). The effect of 0.5% ethanol, the vehicle for the highest coumaphos concentration, is included as a control. (g) Example ACh responses before and after coumaphos (10 μM) application. (h) The time course of the effect of coumaphos on ACh responses in a different KC. Coumaphos (10–50 μM) inhibits ACh responses without significantly changingIM(−1.3±1.5 pA,n=8) or ACh response kinetics, consistent with a lack of AChE inhibition. Figure 6: Coumaphos oxon has a biphasic effect on ACh responses. The effects of coumaphos oxon on baseline I M and ACh responses were investigated under voltage clamp. ( a ) Coumaphos oxon (200 nM) initially potentiates ACh responses (10 min after application), consistent with AChE inhibition. Subsequently, coumaphos oxon evokes a tonic current and inhibits ACh responses (30 min after application). ( b ) The time course of the effect of coumaphos oxon on I M in a different KC. The tonic current develops slowly and is reversed by d-TC, consistent with nAChR activation by accumulated endogenous ACh. ( c ) Mean (±s.e.m.) data showing the biphasic effect (initial potentiation followed by sustained inhibition) of coumaphos oxon ( n =11, * P <0.01, paired t -test) on ACh responses. Included for comparison is the effect of the widely used AChE inhibitor donepezil ( n =7, * P <0.01, paired t -test). ( d ) Mean (±s.e.m.) data showing the effects of coumaphos oxon ( n =11) and donepezil ( n =7) on I M (* P <0.01, paired t -test). Inhibition of ACh responses is associated with an increase in I M (tonic current). ( e ) Mean (±s.e.m.) data showing that the time course of the biphasic effect of coumaphos oxon on ACh responses is dependent on concentration (0.05 μM, n =4; 0.2 μM, n =3; 1 μM, n =4; * P <0.01, unpaired t -test). ( f ) Mean (±s.e.m.) data showing that the parent compound coumaphos inhibits ACh responses at concentrations ≥10 μM (1 μM, n =3; 10 μM, n =5; 50 μM, n =3; * P <0.05, paired t -test). The effect of 0.5% ethanol, the vehicle for the highest coumaphos concentration, is included as a control. ( g ) Example ACh responses before and after coumaphos (10 μM) application. ( h ) The time course of the effect of coumaphos on ACh responses in a different KC. Coumaphos (10–50 μM) inhibits ACh responses without significantly changing I M (−1.3±1.5 pA, n =8) or ACh response kinetics, consistent with a lack of AChE inhibition. Full size image The effects of imidacloprid and coumaphos oxon are additive As honeybees in the United States and parts of Europe are simultaneously exposed to neonicotinoids and coumaphos in the hive [13] , we have examined the effect of their coapplication on KC function. In current-clamped KCs in which coumaphos oxon (10 nM) has produced a stable submaximal depolarization, coapplication of imidacloprid (10–50 nM, n =5) evokes further depolarization ( Fig. 7a ). The magnitude of the additional depolarization evoked by imidacloprid is similar to that evoked by imidacloprid (10–50 nM, n =6) alone ( Fig. 7b ). Thus, cholinergic pesticides with different mechanisms of action have additive effects on KC function. Finally, the effect of combined exposure to field-relevant concentrations of imidacloprid and coumaphos oxon on ACh-evoked depolarizations was determined. Bath application of both imidacloprid (10 nM) and coumaphos oxon (50 nM) evokes a sustained depolarization (of 21±2 mV, n =5) and inhibits ACh responses in current-clamped KCs ( Fig. 7c ). In three of five experiments, a potentiation of ACh responses due to a slowing of their decay was observed before the inhibition ( Fig. 7c ), similar to the effect of coumaphos oxon on ACh responses under voltage clamp ( Fig. 6a ). KCs exposed to nanomolar concentrations of cholinergic pesticides for a prolonged period of time therefore exhibit a reduced responsiveness to ACh as a result of tonic depolarization. 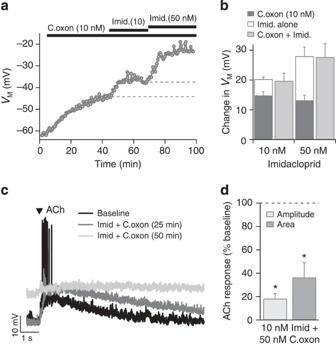Figure 7:Cholinergic pesticides have additive effects on KCVMand inhibit ACh-evoked depolarizations. As honeybees are likely to be exposed to both neonicotinoids and miticides, the effect of coapplication on KC function were determined. (a) Under current clamp, application of coumaphos oxon evokes depolarization of KCVM. Subsequent coapplication of imidacloprid evokes a further concentration-dependent depolarization. (b) Comparison of the sum of the depolarizations evoked by coumaphos oxon and imidacloprid alone (imidacloprid data fromFig. 1e), with the depolarization evoked by the coapplied pesticides (mean±s.e.m.; 10 nM,n=5; 50 nM,n=3). The depolarizations are very similar in magnitude, indicating that the effects of imidacloprid and coumaphos oxon on KC function are additive. (c) The effect of combined pesticide exposure on the response of KCs to ACh was examined under current clamp. Local application of ACh (200 μM, 100 ms) evokes a transient depolarization and burst of APs. Coapplication of imidacloprid (10 nM) plus coumaphos oxon (50 nM) initially slows the decay of ACh responses (25 min after application) due to AChE inhibition. Subsequently, the pesticides evoke sustained depolarization of KCVMand inhibit ACh-evoked responses (50 min after application). (d) Mean (±s.e.m.) data showing the sustained effect of imidacloprid plus coumaphos oxon on the size of ACh-evoked depolarizations (n=5, *P<0.05, pairedt-test). Cholinergic pesticides reduce the responsiveness of KCs to ACh by causing tonic depolarization. Figure 7: Cholinergic pesticides have additive effects on KC V M and inhibit ACh-evoked depolarizations. As honeybees are likely to be exposed to both neonicotinoids and miticides, the effect of coapplication on KC function were determined. ( a ) Under current clamp, application of coumaphos oxon evokes depolarization of KC V M . Subsequent coapplication of imidacloprid evokes a further concentration-dependent depolarization. ( b ) Comparison of the sum of the depolarizations evoked by coumaphos oxon and imidacloprid alone (imidacloprid data from Fig. 1e ), with the depolarization evoked by the coapplied pesticides (mean±s.e.m. ; 10 nM, n =5; 50 nM, n =3). The depolarizations are very similar in magnitude, indicating that the effects of imidacloprid and coumaphos oxon on KC function are additive. ( c ) The effect of combined pesticide exposure on the response of KCs to ACh was examined under current clamp. Local application of ACh (200 μM, 100 ms) evokes a transient depolarization and burst of APs. Coapplication of imidacloprid (10 nM) plus coumaphos oxon (50 nM) initially slows the decay of ACh responses (25 min after application) due to AChE inhibition. Subsequently, the pesticides evoke sustained depolarization of KC V M and inhibit ACh-evoked responses (50 min after application). ( d ) Mean (±s.e.m.) data showing the sustained effect of imidacloprid plus coumaphos oxon on the size of ACh-evoked depolarizations ( n =5, * P <0.05, paired t -test). Cholinergic pesticides reduce the responsiveness of KCs to ACh by causing tonic depolarization. Full size image Here we show that two widely used neonicotinoids and an organophosphate miticide, by modulating the activity of nAChRs, potently affect the neurophysiological properties of KCs. As a result, KCs will be rendered non-functional because of their inability to fire APs or respond appropriately to excitatory synaptic input. KCs are the major neuronal component of the mushroom bodies, which are particularly large in social bees compared with other insects [20] . The effects of cholinergic pesticides on KCs are expected to lead to significant impairment of all cognitive functions that depend on this higher-order brain region, including multisensory integration, associative learning and memory, and spatial orientation [21] , [22] . Consistent with this, sublethal exposure of honeybees to neonicotinoids significantly impairs olfactory learning in laboratory-based studies [38] , [39] , [40] , [41] , and adversely affects navigation and foraging behaviour in the field [7] , [8] , [9] , [10] , [11] . Imidacloprid acts as a partial agonist of nAChRs in cultured honeybee KCs, exhibiting an EC 50 value of 25 ( [18] ) or 0.53 μM [19] . However, cultured KCs are an inadequate model for determining the effect of neonicotinoids on KC functional properties due to changes in the expression of voltage-gated channels and nAChRs, as a result of either the loss of synaptic architecture or normal neuronal activity, or altered developmental expression profiles. For example, cultured KCs show less adaptation in AP firing [29] , which may be related to the absence of Ca 2+ -dependent K + currents from cultured KCs in some studies [25] , [26] , [28] , [29] . The kinetics of ACh-evoked responses appear to differ between KCs in the acutely isolated brain and in culture, and between cultured KCs from pupal and adult honeybees [19] , [24] , [34] . This may result from differences in nAChR desensitization, which is likely to be important for determining the effect of neonicotinoids on KC function [35] . Recordings from KCs in intact honeybee brain are therefore required to provide a mechanistic link between the molecular actions of neonicotinoids and observed behavioural effects. We find that both imidacloprid and clothianidin affect KC excitability at concentrations as low as 10 nM. Although low concentrations of neonicotinoids transiently increase KC excitability, our data indicates that the predominant effect of exposure will be inhibition of AP firing, which is expected to significantly impair mushroom body function. Honeybees are exposed to very high levels of the organophosphate miticide coumaphos in the hive [14] , [42] . The intact brain preparation has enabled us to study the effect of AChE inhibition by coumaphos oxon, the active metabolite of coumaphos, on neuronal function for the first time. Coumaphos oxon is a potent inhibitor of AChE, exhibiting an IC 50 value of 62 nM in honeybee brain ( Fig. 3 ), and producing effects on KC excitability at 10 nM. Coumaphos oxon evokes a slowly developing KC depolarization, due to nAChR activation by accumulated endogenous ACh, causing a transient increase in excitability followed by inhibition of AP firing. The concentration-dependent time course of the biphasic effect of coumaphos oxon on ACh-evoked responses suggests that it will have complex actions on KC function in vivo. Thus, cognitive effects resulting from exposure to coumaphos may range from enhancement to the ablation of learning and memory in honeybees. Indeed, increased learning has been observed in honeybees exposed to other AChE inhibitors [43] , [44] . The balance between enhancement and disruption of learning is expected to be influenced by the level (concentration and duration) of coumaphos exposure and its rate of metabolism to coumaphos oxon, and may be altered for exposure to other organophosphates and in other pollinating insects, such as bumblebees, moths and flies. A critical factor in relating laboratory-based observations of pesticide actions on bee physiology or behaviour to the observed insect pollinator declines is whether the concentration dependence of the observed effects falls within a field-realistic range. Our results suggest that mushroom body dysfunction will result from environmental exposure of honeybees to imidacloprid, clothianidin (which is also the active metabolite of thiamethoxam [45] ) and coumaphos. Significant neuronal effects are evoked by all three cholinergic pesticides at a concentration of 10 nM, which equates to ~2.5 p.p.b. clothianidin, ~2.6 p.p.b. imidacloprid and ~3.6 p.p.b. coumaphos oxon. Imidacloprid levels of up to 28 p.p.b. have been detected in plant flowers and nectar [46] , [47] , [48] , and ingested imidacloprid is rapidly distributed within honeybees, including to the head [49] . Active metabolites such as imidacloprid–olefin, which also evokes KC depolarization due to its activity as a nAChR agonist ( Fig. 2e ) [30] , are detectable in the head for up to 30 h after ingestion [49] . Clothianidin has been found at 3.8–13.3 p.p.b. in dead and dying honeybees collected near the hive entrance in a field study [50] . The miticide coumaphos is found at very high levels in honeybees from treated hives (mean 50.4 p.p.b. [14] , peaking at 0.44–1 p.p.m. one day after treatment [42] ), and coumaphos oxon has been detected at 4.5 p.p.b [14] . The field-relevant effects of coumaphos are likely to be mediated by its oxon metabolite rather than by the direct inhibition of nAChRs that we observed at concentrations ≥10 μM (3.6 p.p.m. ), as although similar coumaphos concentrations are found in hive wax, they are not reached in honeybees [14] , [51] . Furthermore, as coumaphos oxon is an irreversible inhibitor of AChE [52] , its effects on neuronal function are likely to outlast its presence in the brain. The additive effects of imidacloprid and coumaphos oxon on KC function indicate that cholinergic pesticides with different mechanisms of action can interact at the neuronal level. This type of interaction may be of relevance for all classes of pesticide that target neuronal function; for example, the activation of Na + channels by fluvalinate, a pyrethroid miticide, is also expected to enhance the depolarizing effect of neonicotinoids. Importantly, coumaphos, fluvalinate and chlorpyrifos, an agricultural organophosphate pesticide, are the three most prevalent contaminants of hives in the United States [14] , [51] . Both fluvalinate and chlorpyrifos are also widely used in the United Kingdom, where coumaphos is not licensed for use. It is interesting to speculate that the physiological effects of coumaphos identified here may be contributing to the increased honeybee losses observed in the United States: comparative losses in the United States and England have been 35.8%/30.5% (2007–8), 29%/18.7% (2008–9), 42.2%/17.7% (2009–10) and 38.4%/13.6% (2010–11) [53] , [54] , [55] , [56] , [57] . However, it is important to stress that other contributing factors, such as Varroa and the viruses they transmit, Nosema or nutrition have not been considered. There is politically charged debate over whether we should, or could, ban the use of neonicotinoid pesticides, but miticides such as coumaphos may pose a greater risk to honeybee health because of high exposure levels. The emergence of Varroa resistance to both coumaphos and fluvalinate, along with the effectiveness of the organic (oxalic and formic) acids as alternative treatments, suggests that this is one threat to bees that is unnecessary. In summary, our findings show that imidacloprid, clothianidin and coumaphos oxon are potent neuromodulators in the insect brain. We provide a cellular correlate for the effects of neonicotinoids on honeybee cognition and behaviour, and postulate that exposure to multiple cholinergic pesticides will cause enhanced neurotoxicity. An understanding of the neuronal basis of pesticide effects is a prerequisite for developing pest control strategies with greater selectivity for target species. KC electrophysiology Adult worker honeybees ( Apis mellifera mellifera) were anaesthetized on ice and the intact brain isolated while submerged in extracellular solution. Surrounding tissue and membranes were removed by a combination of manual dissection and treatment for 5 min with papain (0.3 mg ml −1 ), L -cysteine (1 mg ml −1 ), collagenase (64 μg ml −1 ) and dispase (0.7 mg ml −1 ) [58] . The removal of covering membranes was necessary to obtain successful whole-cell recordings from KCs. The brain was normally hemisected to reduce animal use, transferred to the recording chamber, secured with a mesh weight and continuously perfused with extracellular solution comprising (in mM) the following: NaCl (140), KCl (5), MgCl 2 (1), CaCl 2 (2.5), NaHCO 3 (4), NaH 2 PO 4 (1.2), HEPES (6) and glucose (14), adjusted to pH 7.4 with NaOH, 326 mOsm [59] . Brain isolation and neuronal recordings were performed at room temperature (18–22 °C). Whole-cell voltage-clamp and current-clamp recordings were obtained from visually identified mushroom body KCs. Patch pipettes (8–10 MΩ) were pulled from borosilicate glass and filled with solution comprising (mM) the following: K-gluconate (110), HEPES (25), KCl (10), MgCl 2 (5), Mg-ATP (3), Na-GTP (0.5) and EGTA (0.5), pH 7.2, 284 mOsm. I M and V M were recorded via an EPC-10 patch-clamp amplifier controlled by Patchmaster software (HEKA). Holding potentials ( V H ) and measured V M were corrected after the experiment for a liquid junction potential of +13 mV. Series resistance ( R S ) and membrane capacitance ( C M ) were calculated from a double-exponential fit of the capacitative current. R S was monitored throughout experiments and recordings were not used if I M or V M changes were accompanied by changes in R S . Transient nAChR-mediated responses were evoked via pressure application (10–20 psi using a Picospritzer II) of ACh (200 μM, 100 ms) from a glass micropipette positioned 25–50 μM from the recorded KC. Antagonists and pesticides were bath-applied via the extracellular solution. ACh-evoked currents were recorded at a V H of −73 mV and quantified by measurement of charge; example currents show the average of four consecutive responses evoked at 30-s intervals. Off-line analysis was performed using IgorPro software (WaveMetrics). Pooled data are expressed as mean±s.e.m. ; n numbers refer to the number of tested KCs for a drug or pesticide, each of which was from a different honeybee. In some current-clamp recordings, two concentrations of the same pesticide were tested; the figure legends provide n numbers for each concentration. Statistical significance was assessed using paired or unpaired Student’s t -tests as appropriate, with P <0.05 considered significant (*). AChE assay Honeybee brains were extracted by dissection and homogenized in PBS. Protein concentrations were determined by the Bradford assay and AChE activity assayed at 14 μg ml −1 . AChE activity was determined using the Ellman assay. AChE inhibitors (at appropriate concentrations) were incubated in honeybee brain lysates for 20 min. Samples were then incubated at room temperature with a reaction mix containing the colour indicator 5′, 5′ Dithiobis (2-nitrobenzoic acid) (286 μM), ACh iodide substrate (0.86 mM) for 30 min and AChE activity monitored by absorbance at 412 nM. AChE activity was normalized to control measurements. IC 50 values were obtained from Hill equation fits of the data from three independent experiments. How to cite this article: Palmer, M.J. et al . Cholinergic pesticides cause mushroom body neuronal inactivation in honeybees. Nat. Commun. 4:1634 doi: 10.1038/ncomms2648 (2013).